Insights into the biomedical effects of carboxylated single-wall carbon nanotubes on telomerase and telomeres Both human telomeric G-rich and C-rich DNA have been considered as specific drug targets for cancer therapy. However, due to i-motif structure instability and lack of specific binding agents, it remains unclear whether stabilization of telomeric i-motif can inhibit telomerase activity. Single-walled carbon nanotubes (SWNTs) have been reported as the first ligand that can selectively stabilize human telomeric i-motif DNA. Here we report that SWNTs can inhibit telomerase activity through stabilization of i-motif structure. The persistence of i-motif and the concomitant G-quadruplex eventually leads to telomere uncapping and displaces telomere-binding proteins from telomere. The dysfunctional telomere triggers DNA damage response and elicits upregulation of p16 and p21 proteins. This is the first example that SWNTs can inhibit telomerase activity and interfere with the telomere functions in cancer cells. These results provide new insights into understanding the biomedical effects of SWNTs and the biological importance of i-motif DNA. Telomeres have important roles in chromosome structural integrity to cap and protect their extremities from illegitimate recombination, degradation and end-to-end fusion [1] . In humans, the telomere is composed of G-rich and C-rich duplex with a single-stranded (ss) 3′-overhang; the G-rich strand can form a four-stranded G-quadruplex structure, and its complementary C-rich strand may adopt intercalated i-motif structures [2] ( Fig. 1a ). The 3′-overhang is either accessible for telomerase extension in an open state or inaccessible in a capped (or closed) conformation that involves the formation of loop motifs, termed as T-loop and D-loop [1] , [3] . Uncapping of the telomere ends by different means leads to telomeric dysfunction characterized by end-to-end fusion, inappropriate recombination, anaphase bridges and G-overhang degradation that either result in apoptosis or senescence [1] , [3] , [4] . 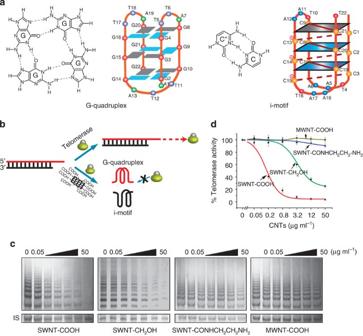Figure 1: SWNTs can inhibit telomerase activityin vitrobased on TRAP-G4 assay. (a) G-quartet and schematic structure of the intramolecular G-quadruplex from human telomere sequence 5′-AG3(T2AG3)3in Na+(left). C·C+base pair and schematic structure of the intramolecular i-motif from human telomere sequence 5′-(C3TA2)3C3T-3′ (right), corresponding complementary strand to 5′-AG3(T2AG3)3. (b) Scheme of inhibition of telomerase activity induced by SWNT-COOH. (c) Inhibition of telomerase activity induced by SWNT-COOH, SWNT-CH2OH, SWNT-CONHCH2CH2NH2and MWNT-COOH in TRAP-G4 assayin vitro. The top panel showed a ladder of amplified extension products stained with 0.2% AgNO3after gel electrophoresis; the black slope corresponds to serial fourfold dilutions of CNTs starting from 0.05 to 50 μg ml−1. IS indicated the bands of internal standard. (d) Telomerase activity was quantitated as the percent of the corresponding control sample containing no CNTs. The mean of three independent experiments with comparable results was shown. Error bars indicate±s.d. Figure 1: SWNTs can inhibit telomerase activity in vitro based on TRAP-G4 assay. ( a ) G-quartet and schematic structure of the intramolecular G-quadruplex from human telomere sequence 5′-AG 3 (T 2 AG 3 ) 3 in Na + (left). C·C + base pair and schematic structure of the intramolecular i-motif from human telomere sequence 5′-(C 3 TA 2 ) 3 C 3 T-3′ (right), corresponding complementary strand to 5′-AG 3 (T 2 AG 3 ) 3 . ( b ) Scheme of inhibition of telomerase activity induced by SWNT-COOH. ( c ) Inhibition of telomerase activity induced by SWNT-COOH, SWNT-CH 2 OH, SWNT-CONHCH 2 CH 2 NH 2 and MWNT-COOH in TRAP-G4 assay in vitro . The top panel showed a ladder of amplified extension products stained with 0.2% AgNO 3 after gel electrophoresis; the black slope corresponds to serial fourfold dilutions of CNTs starting from 0.05 to 50 μg ml −1 . IS indicated the bands of internal standard. ( d ) Telomerase activity was quantitated as the percent of the corresponding control sample containing no CNTs. The mean of three independent experiments with comparable results was shown. Error bars indicate±s.d. Full size image Both human telomeric G-rich and C-rich DNA have been considered as specific drug targets for cancer therapy. In contrast to normal human somatic cells, 85–90% tumor cells express telomerase, an enzyme that stabilizes chromosome ends by adding tandem telomeric DNA repeats to the 3′-overhangs, which is essential for their indefinite proliferative capacities. G-quadruplex formation can inhibit telomerase activity [5] . Many compounds that can stabilize G-quadruplex structure and inhibit telomerase activity have been reported [6] . Along with G-quadruplexes, the biological relevances of C-rich DNA formed i-motif structure have been evidenced by its involvement in human telomeric and centromeric DNA structures and RNA-intercalated structures, and by the discovery of several proteins that bind specifically to C-rich telomeric DNA fragments capable of forming i-motifs [2] , [7] . Most recently, i-motif has also been identified in some oncogene promoter regions, in concert with the G-quadruplex formation on the complementary strand [8] . Although significant progress has been made, because of i-motif structure instability and lack of specific i-motif binding agents, the biological effects of C-rich DNA to form i-motif structure have not been sufficiently clarified [2] , [7] . Especially, it remains unclear whether stabilization of i-motif structure can inhibit telomerase activity. Single-walled carbon nanotubes (SWNTs) have been considered as the leading nanodevice candidate, whose interactions with nucleic acids have attracted much attention. Zheng et al . [9] have shown that a particular sequence of ssDNA self-assembles into a helical structure around individual carbon nanotubes. A piece of double-stranded (ds) DNA wrapped on the surface of a SWNT can serve as sensors in living cells based on the transition of DNA secondary structure from the native, right-handed 'B' form to the alternate, left-handed 'Z' form [10] . A series of DNA interactions with SWNTs have been studied by our group [11] , [12] , [13] , [14] , [15] , [16] , [17] , [18] . We found that SWNTs can destabilize duplex DNA and induce a sequence-dependent DNA B–A transition [11] and can facilitate self-structuring of ssRNA poly(rA) to form A·A + duplex structure [12] . Intriguingly, SWNTs, not multi-walled carbon nanotubes (MWNTs), can selectively stabilize human telomeric i-motif DNA and induce i-motif structure formation by binding to the 5′-end major groove under physiological conditions [13] , [14] , [15] , [16] ( Supplementary Figs S1 and S2 ), and even under molecular crowding conditions [17] . Further studies indicate that SWNTs do not stabilize G-quadruplex DNA and can cause human telomeric duplex to disassociate by forming i-motif and G-quadruplex DNA. This makes SWNTs as the first selective i-motif DNA-binding agent and suitable probe to study the biological function of i-motif both in vitro and in vivo . In this article, we show that SWNTs, not MWNTs, can inhibit telomerase activity both in vitro and in vivo . SWNTs can induce telomere uncapping and removal of telomere-binding protein from telomere, resulting in telomere aberration, DNA damage response and cell growth cessation. Our work will enhance understanding the biomedical effects of SWNTs in cells and the biological function of i-motif DNA in vivo . In vitro inhibition of telomerase activity Although SWNTs do not stabilize G-quadruplex DNA, they can cause human telomeric duplex to disassociate. SWNTs-induced duplex dissociation and i-motif formation will indirectly facilitate the complementary telomeric G-rich strand [13] , [14] , [15] , [16] to fold into G-quadruplex structure, especially under near-physiological conditions of pH and salt concentration [19] ( Fig. 1b ). It is well known that G-quadruplex formation can inhibit telomerase activity. Using a modified TRAP-G4 assay [20] , [21] , [22] , [23] , we explored whether SWNTs could inhibit telomerase activity. As shown in Fig. 1c,d and Supplementary Figure S3 , telomerase activity was significantly inhibited (>80%) by addition of 0.8 μg ml −1 carboxylated SWNTs (SWNT-COOH), and almost complete inhibition was observed at concentrations higher than 3 μg ml −1 . Meanwhile, no inhibition of telomerase substrate internal control (Taq polymerase activity) was observed at concentrations for telomerase activity. Furthermore, only moderate inhibition was observed with hydroxylated SWNTs (SWNT-CH 2 OH), significant inhibition (>80%) appeared only when concentrations used were up to 50 μg ml −1 ( Fig. 1c ). The IC 50 values for SWNT-COOH and SWNT-CH 2 OH on telomerase inhibition were 0.27±0.02 and 7.5±0.25 μg ml −1 , respectively. In contrast, slight or no inhibition was found with aminated SWNTs (SWNT-CONHCH 2 CH 2 NH 2 + ; Fig. 1c,d ). The differences in telomerase inhibition among these functionalized carbon nanotubes (CNTs) can be attributed to their different ability of stabilization and induction of i-motif formation in vitro , which has been related to SWNTs surface charges [13] , [14] , [15] , [16] , [17] . As reported previously, carboxyl-modified SWNTs increased the i-motif Tm by 22 °C. However, the positively charged amino group-modified SWNTs decreased the i-motif Tm by 2 °C [13] . These results indicate that a negatively charged group on the open end of the side wall enhances the interactions with i-motif CC + base pairs by providing favourable electrostatic attractions [11] . These findings are also consistent with our other works that carboxyl- or hydroxyl-modified SWNTs can facilitate polyrA to form A·A + duplex structure at pH 7.0, whereas no such effect was observed with positively charged amino-modified SWNTs [12] . As for carboxylated MWNTs (MWNT-COOH) ( Fig. 1c,d ), no inhibition of telomerase activity was observed. This can be due to the larger diameter of MWNTs compared with SWNTs ( Supplementary Table S1 and Supplementary Fig. S4 ). We have demonstrated that the minor groove of i-motif DNA is too narrow to fit a rigid nanotube (1.1-nm sized SWNTs) and the SWNTs rather bind to the DNA major groove [13] , [14] , [15] , [16] , [17] . However, MWNTs (10–20-nm sized used) are too large to bind to the major groove [15] , so it cannot induce i-motif DNA formation. Taken together, according to the telomerase-inhibition data, telomerase inhibition is related to the different ability of CNTs for stabilization and induction of i-motif formation in vitro . Inhibition of telomerase activity in living cells The intriguing in vitro inhibition results prompted us to investigate whether SWNTs could inhibit telomerase activity in living cancer cells. Increasing evidence has shown that SWNTs can enter cells through the lipid bilayer, and interact with organelles or even localize within the cell nucleus [24] , [25] , [26] . Moreover, it has also been demonstrated that the nature of the functional group on the CNT surface does not determine whether functionalized CNTs are internalized or not [25] . To further determine the localization of SWNTs within cells, we modified the SWNTs with PEG 1500N and labelled with fluorescein isothocyanate (FITC) as described previously [27] ( Supplementary Methods and Supplementary Figs S5–S7 ). As shown in Fig. 2a , after 24 h incubation with SWNT-PEG-FITC, the SWNTs entered the nucleus, and especially localized at telomere, as clarified by the co-localizations with telomere binding protein TRF1, an effective marker for interphase telomeres [1] . We also presented evidences that SWNTs entered the cells through the lysosome pathway and in an energy-dependent manner ( Supplementary Fig. S7 ). Keeping these in mind, we explored whether SWNTs could still inhibit telomerase activity in living cancer cells. 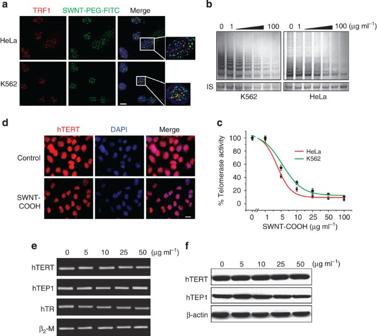Figure 2: SWNTs can localize at telomeres and inhibit telomerase activity in living cancer cells. (a) SWNTs localizes at telomere in K562 and HeLa cells evidenced by the co-localizations with telomere marker TRF1 protein. K562 and HeLa cells were incubated with SWNT-PEG-FITC (green) for 24 h and co-stained with anti-TRF1 antibody (red). White rectangles in merged pictures were enlarged as shown in right, yellow dots indicated the co-localization signals. Scale bar equals 10 μM. (b) Telomerase activity inhibition induced by carboxylated SWNTs in human K562 and HeLa cells. Cells were treated with increasing concentrations of carboxylated SWNTs for 6 days, CHAPS extract was prepared and equivalent amounts of protein (500 ng) were subjected to a standard TRAP assay. The position of the internal standard was indicated as IS. (c) Telomerase activity was quantitated as the percent of the corresponding control sample containing no CNTs. The mean of three independent experiments with comparable results was shown. Error bars indicate±s.d. (d) SWNT-COOH treatment does not induce the change of localization of hTERT in K562 cells. After treatment with SWNT-COOH for 1 week, K562 cells were stained with anti-hTERT antibody (red) and the nucleus were visualized with DAPI staining (blue), and the merged image is shown in right. Scale bar equals 20 μM. (e) SWNT-COOH doses not induce the change of expression of hTERT, hTEP1 and hTR at mRNA levels by using semi-quantitative RT–PCR assay. β2-M was used as loading control. (f) SWNT-COOH doses not induce the alternation of expression of hTERT and hTEP1 at protein levels. After 1 week of treatment, the protein was extracted and subjected to western blotting, then probed with anti-hTERT and anti-hTEP1 antibodies. β-actin was used as loading control. Figure 2: SWNTs can localize at telomeres and inhibit telomerase activity in living cancer cells. ( a ) SWNTs localizes at telomere in K562 and HeLa cells evidenced by the co-localizations with telomere marker TRF1 protein. K562 and HeLa cells were incubated with SWNT-PEG-FITC (green) for 24 h and co-stained with anti-TRF1 antibody (red). White rectangles in merged pictures were enlarged as shown in right, yellow dots indicated the co-localization signals. Scale bar equals 10 μM. ( b ) Telomerase activity inhibition induced by carboxylated SWNTs in human K562 and HeLa cells. Cells were treated with increasing concentrations of carboxylated SWNTs for 6 days, CHAPS extract was prepared and equivalent amounts of protein (500 ng) were subjected to a standard TRAP assay. The position of the internal standard was indicated as IS. ( c ) Telomerase activity was quantitated as the percent of the corresponding control sample containing no CNTs. The mean of three independent experiments with comparable results was shown. Error bars indicate±s.d. ( d ) SWNT-COOH treatment does not induce the change of localization of hTERT in K562 cells. After treatment with SWNT-COOH for 1 week, K562 cells were stained with anti-hTERT antibody (red) and the nucleus were visualized with DAPI staining (blue), and the merged image is shown in right. Scale bar equals 20 μM. ( e ) SWNT-COOH doses not induce the change of expression of hTERT, hTEP1 and hTR at mRNA levels by using semi-quantitative RT–PCR assay. β 2 -M was used as loading control. ( f ) SWNT-COOH doses not induce the alternation of expression of hTERT and hTEP1 at protein levels. After 1 week of treatment, the protein was extracted and subjected to western blotting, then probed with anti-hTERT and anti-hTEP1 antibodies. β-actin was used as loading control. Full size image K562 and HeLa cells were cultured in the presence of SWNTs at concentrations ranging from 1 to 100 μg ml −1 . After 6 days, cells were lysed and telomerase activity was assessed in the extracts with a conventional tartarate-resistant acid phosphatase (TRAP) assay [28] . As shown in Fig. 2b,c , a clear concentration-dependent loss of telomerase activity was observed. IC 50 values of SWNTs for telomerase inhibition in K562 and HeLa cells were 10.2±0.8 and 7.5±0.45 μg ml −1 , respectively. The extent of inhibition of telomerase activity by SWNTs in whole cells paralleled the relative potency on telomerase inhibition in vitro . In addition, the inhibition of telomerase activity by SWNTs was also time-dependent. The inhibitory efficiency reached maximum on day 9 after treatment, afterwards, entered the plateau phase ( Supplementary Fig. S8 ). Furthermore, we also investigated the effects of different functionalized CNTs on intracellular telomerase activity inhibition to see whether the differences in size and surface charges of different functionalized SWNTs and MWNTs on i-motif stabilization and telomerase activity inhibition in vitro could still exist in living cells. Their IC 50 values were summarized in Supplementary Table S2 . The same trend was observed: carboxylated SWNTs showed strong inhibition, hydroxylated SWNTs had moderate inhibition, slight or no inhibition for aminated SWNTs and carboxylated MWNTs. Moreover, based on the fact that intracellular environments are highly crowded with various biomolecules, therefore, in vitro studies under molecular-crowding conditions will provide important information on how biomolecules behave in cells [17] , [29] . We have shown that SWNTs can induce i-motif formation under cell-mimic crowding conditions [17] . In addition to the various interactions of DNA bases and backbone with SWNTs, such as hydrophobic and van der Waals interactions, the favourable electrostatic interactions between the positively charged C–C + base pairs and the carboxyl groups on low MW and massive MW SWNTs can change the p K a of the C–C + base pairs and induce i-motif formation, and molecular crowding can further stabilize i-motif and cause more water molecules to be released [17] . Besides, we have demonstrated that SWNTs can enter the living cells in an energy and lysosome-dependent pathway, and pierce into the nucleus ( Supplementary Fig. S7 ), consistent with previous reports [24] , [25] , [26] . More direct evidence for the telomeric localization of SWNT in the nuclei has also been provided ( Fig. 2a ). Sugimoto and co-workers [29] have demonstrated that molecular crowding can destabilize duplex DNA and enhance G-quadruplex stability. These provide further support that SWNTs can stabilize human telomeric i-motif DNA and concomitantly induce G-quadruplex formation, which has been evidenced [13] , [16] , and then inhibit telomerase activity in cancer cells. Furthermore, we provided evidences that the inhibition of telomerase activity induced by SWNTs was not associated with the translocation of telomerase or the alteration of its expression ( Fig. 2d–f ; Supplementary Fig. S9 ). On the basis of these results, carboxylated SWNTs showed the best inhibitory effect on telomerase activity both in vitro and in living cells. Next, we further studied how carboxylated SWNTs influenced cell proliferation, telomere structure and function. Cell growth suppression and DNA-damage response The acute cytotoxic effects of carboxylated SWNTs in short-term cultures (3 and 6 days) were first assessed by using the XTT assay [30] and Trypan blue exclusion assay in K562 and HeLa cells. As shown in Supplementary Figure S10 , we did not observe any acute toxicity on both K562 and HeLa cells after 3 and 6 days of treatment with concentrations up to 100 μg ml −1 . These were consistent with other reports [31] . The non-acute toxicity induced by carboxylated SWNTs can be attributed to the removal of metal catalysts from SWNTs after mixed-acid treatment, which has also been verified in our previous studies [32] . We further characterized the growth kinetics of cells with carboxylated SWNTs in long-term cultures by assessing the effects on population doublings as our previously described [30] . In this assay, 25 and 50 μg ml −1 were employed, at which concentration telomerase activity could be inhibited but without acute growth inhibitory effect [30] . As shown in Fig. 3a , the decrease in cell proliferation was first observed after 2 weeks of treatment, followed by complete growth arrest after additional 1 week, which was associated with massive cell death, as shown by the apparent decrease in population doubling number between two seedings. To further determine the growth suppression induced by SWNTs was telomerase activity-dependent or telomere structure-dependent, growth curve for transfection of 2′- O -MeRNA, a common telomerase inhibitor [33] or transfection with TRF2 ΔBΔM gene (basic/myb domain defection), which would result in the dysfunctional telomere [34] , was also performed. As shown in Supplementary Figure S11 , transfection of 2′- O -MeRNA for 72 h in HeLa cells caused dose-dependent decrease of telomerase activity with IC 50 =0.11±0.012 μM, and 0.45 μM for 80% inhibition of telomerase activity was used for further experiments. However, transfection of TRF2 ΔBΔM for up to 12 days did not affect the telomerase activity, in agreement with previous reports [34] . Furthermore, the stable expression of TRF2 ΔBΔM in K562 and HeLa cells was confirmed by the immunoblotting targeting the fused myc-tag ( Supplementary Fig. S12 ), whereas transfection with empty vector was almost identical with the untreated groups (data not shown). Transfection with 2′- O -MeRNA did not induce growth arrest in both HeLa and K562 cells for up to 3 weeks ( Fig. 3a ); however, significant growth suppression was observed after 2 weeks of transfection with TRF2 ΔBΔM ( Fig. 3a ), similar to the treatment with SWNTs, suggesting that the cell growth inhibition induced by SWNTs was telomere structure-dependent but not telomerase activity dependent. 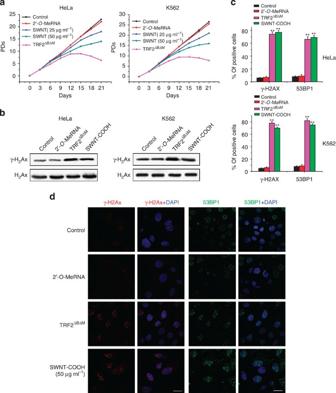Figure 3: Growth suppression induced by SWNT-COOH associates with the production of DNA-damage response. (a) Proliferation curves of HeLa and K562 cells treated with 2′-O-MeRNA, SWNT-COOH (25 and 50 μg ml−1, respectively.) or transfected with TRF2ΔBΔMAt the indicated times, cells were counted and the population doublings (PDs) were determined. (b) Western blot analysis of γ-H2AX in K562 and HeLa cells treated with 2′-O-MeRNA, SWNT-COOH (50 μg ml−1) or transfected with TRF2ΔBΔMfor 2 weeks. The levels of H2AX were used as loading control. (c) Percentage of cells containing γ-H2AX and 53BP1 foci in K562 and HeLa cells treated with 2′-O-MeRNA, SWNT-COOH (50 μg ml−1) or transfected with TRF2ΔBΔMfor 2 weeks. γ-H2AX and 53BP1 foci were quantified using mouse monoclonal antibodies. On average, more than 200 cells were screened in three independent experiments. Error bars indicate s.d. **P<0.001, two-tailed Student'st-test. (d) Representative immunofluorescence images of γ-H2AX and 53BP1 foci in HeLa cells treated with 2′-O-MeRNA, SWNT-COOH (50 μg ml−1) or transfected with TRF2ΔBΔMfor 2 weeks. Scale bar equals 20 μM. Figure 3: Growth suppression induced by SWNT-COOH associates with the production of DNA-damage response. ( a ) Proliferation curves of HeLa and K562 cells treated with 2′- O -MeRNA, SWNT-COOH (25 and 50 μg ml −1 , respectively.) or transfected with TRF2 ΔBΔM At the indicated times, cells were counted and the population doublings (PDs) were determined. ( b ) Western blot analysis of γ-H2AX in K562 and HeLa cells treated with 2′- O -MeRNA, SWNT-COOH (50 μg ml −1 ) or transfected with TRF2 ΔBΔM for 2 weeks. The levels of H2AX were used as loading control. ( c ) Percentage of cells containing γ-H2AX and 53BP1 foci in K562 and HeLa cells treated with 2′- O -MeRNA, SWNT-COOH (50 μg ml −1 ) or transfected with TRF2 ΔBΔM for 2 weeks. γ-H2AX and 53BP1 foci were quantified using mouse monoclonal antibodies. On average, more than 200 cells were screened in three independent experiments. Error bars indicate s.d. ** P <0.001, two-tailed Student's t -test. ( d ) Representative immunofluorescence images of γ-H2AX and 53BP1 foci in HeLa cells treated with 2′- O -MeRNA, SWNT-COOH (50 μg ml −1 ) or transfected with TRF2 ΔBΔM for 2 weeks. Scale bar equals 20 μM. Full size image Previous reports have shown that growth suppression induced by telomere-targeting agents often associates with the telomere dysfunction and production of DNA-damage response [6] . Therefore, we investigated whether the treatment with SWNTs would induce the production of DNA-damage response. As shown in Fig. 3b , strong phosphorylation of γ-H2AX after 2-weeks treatment with SWNTs (50 μg ml −1 ), which was a hallmark of DNA double-strand break response [1] , [35] , was observed, which was also confirmed by the immunofluorescence for γ-H2AX and 53BP1, another DNA-damage response factor [1] , [35] . More γ-H2AX- and 53BP1-positive cells were observed after treatment with SWNTs (50 μg ml −1 ) compared with untreated groups ( Fig. 3c,d , P <0.001). Meanwhile, transfection with TRF2 ΔBΔM also induced significant upregulation of γ-H2AX, and more γ-H2AX and 53BP1 foci in cells [1] , [35] ; however, transfection with 2′- O -MeRNA did not exhibit these effects. DNA-damage response triggered by SWNTs occurred at telomere To verify whether γ-H2AX and 53BP1 were activated at telomeres, double immunofluorescence experiments were performed in HeLa cells. Confocal microscopy revealed that most of the γ-H2AX foci and 53BP1 foci induced by SWNTs colocalized with TRF1 ( Fig. 4a–c ), forming the so-called telomere dysfunction-induced foci (TIFs) [1] , [35] . Quantitative analysis indicated that SWNTs significantly increased the percentage of cells with more than four γ-H2AX/TRF1 or 53BP1/TRF1 colocalizations (the percentage of TIFs-positive cells reached about 60% upon treatment; P <0.01), with a mean of ca . six TIFs per nucleus ( Fig. 4b,c ). Notably, an important fraction of the damage response was not colocalized at telomeres. Analysis of human genome composition has identified that many i-motif and G-quadruplex-forming sequences are located outside telomeres [36] . Therefore, it is possible that SWNTs can also interact with other i-motif and G-quadruplex targets [6] . These results were confirmed by quantitative reverse-transcription PCR (qRT–PCR)-based chromatin immunoprecipitation (ChIP) as described previously [37] . The ChIP assay showed that γ-H2AX and 53BP1 associated to telomeres in SWNT-treated cells ( Fig. 4d ). Telomere damage caused by SWNTs appeared to be very potent, as the percentage of cells with more than four TIFs approached that measured in cells expressing the TRF2 ΔBΔM allele [35] ( Fig. 4a–c ). However, no or slight telomeric DNA-damage response was found in 2′- O -MeRNA-transfected cells. These telomere-based DNA damage responses have also been reported for some G-quadruplex interactive agents [6] , [37] . 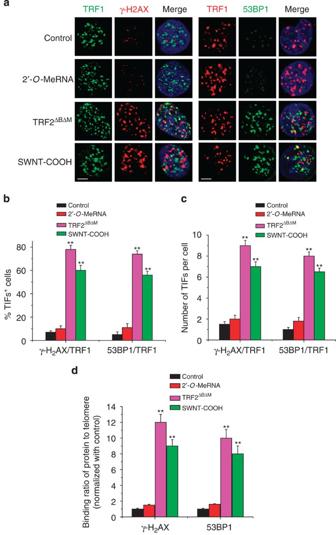Figure 4: DNA-damage response triggered by SWNT-COOH occurred at telomeres. (a) HeLa cells expressing TRF2ΔBΔMor treated with either 2′-O-MeRNA or SWNT-COOH (50 μg ml−1) for 2 weeks were fixed and processed for immunofluorescence using antibodies against γ-H2AX (red)/TRF1 (green) or 53BP1 (green)/TRF1 (red), respectively. Representative confocal images were shown. Scale bar equals 5 μM. (b) TIF index, defined as foci of DNA-damage response factors that coincided with TRF1, was calculated as the percentage of TIF-positive cells in HeLa cells expressing TRF2ΔBΔMor treated with either 2′-O-MeRNA or SWNT-COOH (50 μg ml−1). Cells with four or more γ-H2AX/TRF1or 53BP1/TRF1 foci were scored as TIF-positive. The mean of three independent experiments was reported. Error bars indicate s.d. **P<0.001, two-tailed Student'st-test. (c) Average number of TIFs per nucleus in HeLa cells expressing TRF2ΔBΔMor treated with either 2′-O-MeRNA or SWNT-COOH (50 μg ml−1). The mean of three independent experiments with comparable results was shown. Error bars indicated±s.d. **P<0.005, two-tailed Student'st-test. (d) Binding of γ-H2AX and 53BP1 was examined by ChIP assay and detected by qRT–PCR amplification of the telomeric region in HeLa cells expressing TRF2ΔBΔMor treated with either 2′-O-MeRNA or SWNT-COOH (50 μg ml−1). Data represented triplicate ChIP experiments, each with technical triplicates of qRT–PCR; **P<0.01 as compared with controls. Figure 4: DNA-damage response triggered by SWNT-COOH occurred at telomeres. ( a ) HeLa cells expressing TRF2 ΔBΔM or treated with either 2′- O -MeRNA or SWNT-COOH (50 μg ml −1 ) for 2 weeks were fixed and processed for immunofluorescence using antibodies against γ-H 2 AX (red)/TRF1 (green) or 53BP1 (green)/TRF1 (red), respectively. Representative confocal images were shown. Scale bar equals 5 μM. ( b ) TIF index, defined as foci of DNA-damage response factors that coincided with TRF1, was calculated as the percentage of TIF-positive cells in HeLa cells expressing TRF2 ΔBΔM or treated with either 2′- O -MeRNA or SWNT-COOH (50 μg ml −1 ). Cells with four or more γ-H2AX/TRF1or 53BP1/TRF1 foci were scored as TIF-positive. The mean of three independent experiments was reported. Error bars indicate s.d. ** P <0.001, two-tailed Student's t -test. ( c ) Average number of TIFs per nucleus in HeLa cells expressing TRF2 ΔBΔM or treated with either 2′- O -MeRNA or SWNT-COOH (50 μg ml −1 ). The mean of three independent experiments with comparable results was shown. Error bars indicated±s.d. ** P <0.005, two-tailed Student's t -test. ( d ) Binding of γ-H2AX and 53BP1 was examined by ChIP assay and detected by qRT–PCR amplification of the telomeric region in HeLa cells expressing TRF2 ΔBΔM or treated with either 2′- O -MeRNA or SWNT-COOH (50 μg ml −1 ). Data represented triplicate ChIP experiments, each with technical triplicates of qRT–PCR; ** P <0.01 as compared with controls. Full size image Telomere uncapping induced by carboxylated SWNTs It has been hypothesized that the induction of quadruplex structures at the telomere may result in alterations of telomere capping, which have been validated during the treatment with G-quadruplex-binding ligands [37] , [38] , [39] , and the alterations have been evidenced by the formation of anaphase bridges, micronuclei and telomere fusion [37] , [38] , [39] . Next, we explored whether telomeric quadruplex formation induced by SWNTs could interfere with telomere integrity and induce formation of anaphase bridges. Telomere status was analysed in HeLa cells by staining of nuclei with DAPI (4′,6-diamidino-2-phenylindole), performed on day 6 after treatment, and revealed that cells treated with SWNTs displayed typical images of anaphase bridges and micronuclei, which indicated telomere uncapping ( Fig. 5a ). Evidently, the anaphase bridge usually co-existed with micronuclei. Similar results were obtained in TRF2 ΔBΔM -expressing cells [34] ( Fig. 5a ). These results may also provide the possible explanation for the genotoxicity induced by SWNTs [40] . Furthermore, metaphases spreads in treated groups were also prepared and stained with DAPI and Giemsa, respectively. As shown in Fig. 5b,c , remarked telomere fusion was observed in SWNTs-treated and TRF2 ΔBΔM -expressing cells [34] ( P <0.001), indicating the alteration of telomere structure. However, transfection with 2′- O -MeRNA did not induce these multiple cytogenetic aberrations. Moreover, to directly label the unprotected telomere, a terminal deoxytransferase (TdT) assay that added cy3-conjugated deoxyuridine to naked telomere ends was applied [41] . The TdT–cy3 assay did not detect specific nuclear staining in untreated and 2′- O -MeRNA-transfected cells. However, in SWNTs-treated cells, ~75% of TdT signals colocalized with telomeres and ~80% for TRF2 ΔBΔM -expressing cells, indicative of robust telomere uncapping ( Fig. 5d–f ). Taken together, these results demonstrated for the first time that carboxylated SWNTs can induce telomere uncapping and expose chromosomal termini to the DNA-damage pathway. 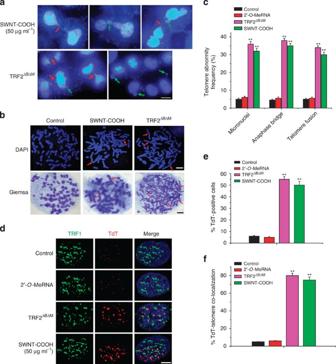Figure 5: Telomere uncapping induced by carboxylated SWNTs. (a) Representative images of anaphase bridges and micronuclei in HeLa cells treated for 6 days with carboxylated SWNTs (50 μg ml−1) or transfected with TRF2ΔBΔMwere shown. Cells were stained with DAPI and images were recorded. Red arrow indicated bridge formation, and green arrow indicated micronuclei formation. Anaphase bridges and micronuclei often co-existed in treated cells. Scale bar equals 10 μM. (b) Telomere fusion induced by carboxylated SWNTs or transfection with TRF2ΔBΔMmetaphase spreads were stained with DAPI or Giemsa, respectively. Scale bar equals 10 μM. (c) The frequency of telomere instability was calculated as the ratio between cells exhibiting anaphase bridges/micronuclei and the total number of anaphase cells (at least 50 anaphase cells were examined). Telomeric fusion frequency was calculated as total number of telomeric fusions/total number of metaphases. The data represented the means of four independent experiments with s.d. **P<0.001. (d) SWNT-COOH induced accessible telomere ends. TRF1 (green) were used to detect telomeres, whereas TdT-cy3 (red) was used as a marker of uncapped telomeres in HeLa cells treated with carboxylated SWNTs, 2′-O-MeRNA or transfection with TRF2ΔBΔMmerged signals were shown in the right. Scale bar equals 5 μM. (e) Quantification of the percentage of TdT-cy3-positive cells in SWNT-COOH, 2′-O-MeRNA or TRF2ΔBΔM-treated cells. (f) Quantification of the percentage of colocalization of telomeric signals with TdT-cy3 signals in SWNT-COOH, 2′-O-MeRNA or TRF2ΔBΔM-treated cells. In panelseandf, a minimum of 100 nuclei was scored, and error bars represented s.d. **P<0.001. Figure 5: Telomere uncapping induced by carboxylated SWNTs. ( a ) Representative images of anaphase bridges and micronuclei in HeLa cells treated for 6 days with carboxylated SWNTs (50 μg ml −1 ) or transfected with TRF2 ΔBΔM were shown. Cells were stained with DAPI and images were recorded. Red arrow indicated bridge formation, and green arrow indicated micronuclei formation. Anaphase bridges and micronuclei often co-existed in treated cells. Scale bar equals 10 μM. ( b ) Telomere fusion induced by carboxylated SWNTs or transfection with TRF2 ΔBΔM metaphase spreads were stained with DAPI or Giemsa, respectively. Scale bar equals 10 μM. ( c ) The frequency of telomere instability was calculated as the ratio between cells exhibiting anaphase bridges/micronuclei and the total number of anaphase cells (at least 50 anaphase cells were examined). Telomeric fusion frequency was calculated as total number of telomeric fusions/total number of metaphases. The data represented the means of four independent experiments with s.d. ** P <0.001. ( d ) SWNT-COOH induced accessible telomere ends. TRF1 (green) were used to detect telomeres, whereas TdT-cy3 (red) was used as a marker of uncapped telomeres in HeLa cells treated with carboxylated SWNTs, 2′- O -MeRNA or transfection with TRF2 ΔBΔM merged signals were shown in the right. Scale bar equals 5 μM. ( e ) Quantification of the percentage of TdT-cy3-positive cells in SWNT-COOH, 2′- O -MeRNA or TRF2 ΔBΔM -treated cells. ( f ) Quantification of the percentage of colocalization of telomeric signals with TdT-cy3 signals in SWNT-COOH, 2′- O -MeRNA or TRF2 ΔBΔM -treated cells. In panels e and f , a minimum of 100 nuclei was scored, and error bars represented s.d. ** P <0.001. Full size image SWNTs induce displacement of telomere-binding proteins To determine the cause of telomere uncapping, we investigated the effect of SWNTs on the localization of TRF2 and POT1, two telomeric proteins that can induce telomere dysfunction and evoke DNA-damage signaling when their levels are reduced at telomeres [1] , [34] , [35] . Furthermore, we also studied the effect of SWNTs on the localization of PCBP1 (poly-(C) binding protein 1) at telomere, which has been identified as a specific telomere C-rich strand binding protein, and may have an important role in telomere maintenance [42] , [43] . Confocal microscopy showed that SWNTs specifically delocalized TRF2, POT1 and PCBP1 from TRF1 foci in HeLa cells after 2 weeks of treatment ( Fig. 6a ). Quantitative analysis indicated that the percentage of nuclei with more than four TRF2/TRF1, POT1/TRF1 or PCBP1/TRF1 co-localizations was markedly reduced in cells exposed to SWNTs ( Fig. 6b,c ). To confirm the results, we performed qRT–PCR-based telomeric ChIP assay as described above. As expected, SWNTs significantly reduced the binding of TRF2, POT1 and PCBP1 to the telomere, without affecting the association of TRF1 to the telomere, consistent with the immunofluorescence results ( Fig. 6d ). We also provided evidences that the removal of TRF2, POT1 and PCBP1 from telomere was not associated with the change of expression of these proteins ( Fig. 6e ). Furthermore, we investigated the effect of SWNTs on telomeric G-overhang length and the total telomere length by using hybridization protection assay (HPA) [38] , [44] . As shown in Fig. 6f , SWNTs significantly reduced the telomeric G-overhang length after 2 weeks of treatment ( P <0.01), whereas the total telomere length did not change. All these similar results were also obtained in TRF2 ΔBΔM -expressing cells, which accorded with previous reports [1] , [34] , [35] . However, cells transfected with 2′- O -MeRNA did not show these effects, except the slight reduction of telomeric G-overhang length after 2 weeks of treatment ( P >0.05). 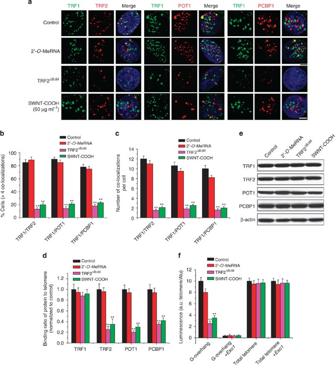Figure 6: SWNTs specifically delocalize TRF2, POT1 and PCBP1 from telomeres and induce telomeric 3′-overhang degradation. (a) HeLa cells expressing TRF2ΔBΔMor treated with either 2′-O-MeRNA or SWNT-COOH (50 μg ml−1) were double stained with the indicated antibodies. Representative confocal images showing merged TRF1 (green) with TRF2, POT1 or PCBP1 (red) staining in untreated and treated cells. Scale bar equals 5 μM. (b) Percentages of cells with more than four colocalizations per nucleus of TRF1/TRF2, TRF1/POT1 or TRF1/PCBP1. The mean of three independent experiments with comparable results was shown. Error bars indicated s.d. **P<0.005. (c) Average number of colocalizations per nucleus in HeLa cells expressing TRF2ΔBΔMor treated with either 2′-O-MeRNA or SWNT-COOH (50 μg ml−1). The mean of three independent experiments with comparable results was shown. Error bars indicated±s.d. **P<0.005, two-tailed Student'st-test. (d) Binding of TRF1, TRF2, POT1 or PCBP1 was examined by ChIP assay and detected by qRT–PCR amplification of the telomeric region in HeLa cells expressing TRF2ΔBΔMor treated with either 2′-O-MeRNA or SWNT-COOH (50 μg ml−1). Data represented triplicate ChIP experiments, each with technical triplicates of qRT–PCR; **P<0.01 as compared with controls. (e) Expression of TRF1, TRF2, POT1 and PCBP1 in HeLa cells expressing TRF2ΔBΔMor treated with either 2′-O-MeRNA or SWNT-COOH (50 μg ml−1). β-actin was used as loading control. (f) Hybridization protection assay (HPA) was performed on genomic DNA isolated from HeLa cells expressing TRF2ΔBΔMor treated with either 2′-O-MeRNA or SWNT-COOH (50 μg ml−1) to assess the length of G-overhang and total telomere length.ExoInuclease digestion was used to assess integrity of the 3′-overhang. Luminescence intensity in arbitrary units (AU) was normalized againstAluprobe. The mean of three independent experiments with comparable results was shown. Error bars indicated±s.d., **P<0.01, two-tailed Student'st-test. Figure 6: SWNTs specifically delocalize TRF2, POT1 and PCBP1 from telomeres and induce telomeric 3′-overhang degradation. ( a ) HeLa cells expressing TRF2 ΔBΔM or treated with either 2′- O -MeRNA or SWNT-COOH (50 μg ml −1 ) were double stained with the indicated antibodies. Representative confocal images showing merged TRF1 (green) with TRF2, POT1 or PCBP1 (red) staining in untreated and treated cells. Scale bar equals 5 μM. ( b ) Percentages of cells with more than four colocalizations per nucleus of TRF1/TRF2, TRF1/POT1 or TRF1/PCBP1. The mean of three independent experiments with comparable results was shown. Error bars indicated s.d. ** P <0.005. ( c ) Average number of colocalizations per nucleus in HeLa cells expressing TRF2 ΔBΔM or treated with either 2′- O -MeRNA or SWNT-COOH (50 μg ml −1 ). The mean of three independent experiments with comparable results was shown. Error bars indicated±s.d. ** P <0.005, two-tailed Student's t -test. ( d ) Binding of TRF1, TRF2, POT1 or PCBP1 was examined by ChIP assay and detected by qRT–PCR amplification of the telomeric region in HeLa cells expressing TRF2 ΔBΔM or treated with either 2′- O -MeRNA or SWNT-COOH (50 μg ml −1 ). Data represented triplicate ChIP experiments, each with technical triplicates of qRT–PCR; ** P <0.01 as compared with controls. ( e ) Expression of TRF1, TRF2, POT1 and PCBP1 in HeLa cells expressing TRF2 ΔBΔM or treated with either 2′- O -MeRNA or SWNT-COOH (50 μg ml −1 ). β-actin was used as loading control. ( f ) Hybridization protection assay (HPA) was performed on genomic DNA isolated from HeLa cells expressing TRF2 ΔBΔM or treated with either 2′- O -MeRNA or SWNT-COOH (50 μg ml −1 ) to assess the length of G-overhang and total telomere length. ExoI nuclease digestion was used to assess integrity of the 3′-overhang. Luminescence intensity in arbitrary units (AU) was normalized against Alu probe. The mean of three independent experiments with comparable results was shown. Error bars indicated±s.d., ** P <0.01, two-tailed Student's t -test. Full size image Cell cycle arrest, apoptosis and senescence evoked by SWNTs Furthermore, we explored whether telomere dysfunction induced by carboxylated SWNTs resulted in cell cycle arrest, apoptosis or senescence. We first analysed the percentage of cells in different phases of the cell cycle. As shown in Fig. 7a , on day 14, SWNTs induced significant accumulation of cells in the G 0 –G 1 phase and concomitant decrease in the S phase ( P <0.01). In contrast, transfection with TRF2 ΔBΔM induced G 2 –M phase arrest, in agreement with previous reports [1] . However, transfection with 2′- O -MeRNA did not induce the alteration of cell cycle distribution. Moreover, on day 21, the cells treated with SWNTs showed strong perturbation of the cell cycle and a fraction of cell population resided to the sub-G1 compartment, indicative of apoptotic cells. Similar cell cycle arrest has been reported during the treatment with G-quadruplex-binding ligand, telomestatin, in OM9;22 cells [45] . 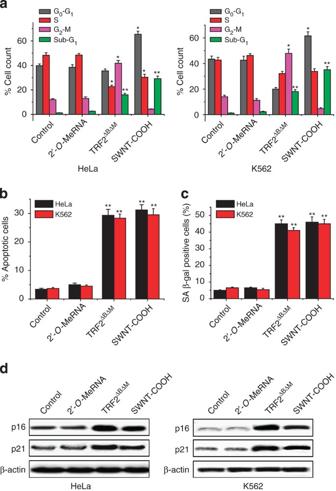Figure 7: Cell cycle arrest, apoptosis and senescence evoked by carboxylated SWNTs-induced telomere dysfunction. (a) Cell cycle arrest induced by carboxylated SWNTs in K562 and HeLa cells. Two weeks after treatment with SWNTs, cells were collected and stained with propidium iodide (PI); DNA content was determined by flow cytometry. The percentages of cells undergoing apoptosis (sub-G1%) were expressed with respect to the total number of cells. This assay was performed in triplicate. *P<0.05, **P<0.01. (b) Apoptotic cell death induced by carboxylated SWNTs in K562 and HeLa cells. Three weeks after treatment with SWNTs, cells were collected and stained with PI and Annexin V–FITC, Annexin V-positive/PI-negative cells were measured by flow cytometry. This experiment was repeated three times. **P<0.001. (c) Expression of senescence-associated β-galactosidase (SA-β-gal) in K562 and HeLa cells after continuous treatment with carboxylated SWNTs for 3 weeks. This assay was performed in triplicate. The senescent cells were counted under an inverted microscope in five random fields. **P<0.001. (d) Upregulation of p16 and p21 proteins induced by carboxylated SWNTs. After K562 and HeLa cells were treated with SWNT-COOH (50 μg ml−1), 2′-O-MeRNA or transfection with TRF2ΔBΔMfor 3 weeks, cells were lysed and separated on 10% SDS–PAGE, and probed with anti-p16INK4aand anti-p21WAF1primary antibody, respectively. Immunoblotting for β-actin was also performed to verify equivalent protein loading. Each experiment has been repeated three times. Figure 7: Cell cycle arrest, apoptosis and senescence evoked by carboxylated SWNTs-induced telomere dysfunction. ( a ) Cell cycle arrest induced by carboxylated SWNTs in K562 and HeLa cells. Two weeks after treatment with SWNTs, cells were collected and stained with propidium iodide (PI); DNA content was determined by flow cytometry. The percentages of cells undergoing apoptosis (sub-G1%) were expressed with respect to the total number of cells. This assay was performed in triplicate. * P <0.05, ** P <0.01. ( b ) Apoptotic cell death induced by carboxylated SWNTs in K562 and HeLa cells. Three weeks after treatment with SWNTs, cells were collected and stained with PI and Annexin V–FITC, Annexin V-positive/PI-negative cells were measured by flow cytometry. This experiment was repeated three times. ** P <0.001. ( c ) Expression of senescence-associated β-galactosidase (SA-β-gal) in K562 and HeLa cells after continuous treatment with carboxylated SWNTs for 3 weeks. This assay was performed in triplicate. The senescent cells were counted under an inverted microscope in five random fields. ** P <0.001. ( d ) Upregulation of p16 and p21 proteins induced by carboxylated SWNTs. After K562 and HeLa cells were treated with SWNT-COOH (50 μg ml −1 ), 2′- O -MeRNA or transfection with TRF2 ΔBΔM for 3 weeks, cells were lysed and separated on 10% SDS–PAGE, and probed with anti-p16 INK4a and anti-p21 WAF1 primary antibody, respectively. Immunoblotting for β-actin was also performed to verify equivalent protein loading. Each experiment has been repeated three times. Full size image Besides, we also observed SWNTs-induced apoptosis and senescence. Annexin V assay [18] was performed in K562 and HeLa cells to assess apoptosis after treatment with SWNTs for 21 days. As shown in Fig. 7b , apoptosis occurred after exposure to SWNTs, consistent with the sub-G 1 quantification in the cell cycle analysis. The induction of apoptosis resulted from the inability of cells to pass the G 1 /S checkpoints. Moreover, the apoptosis was also accompanied by the occurrence of a senescence phenotype: large cell size, vacuolated cytoplasm and β-galactosidase activity [30] . As shown in Fig. 7c , marked increase in the percentage of senescent cells was observed in 50 μg ml −1 SWNTs-treated cells ( P <0.001). Similarly, remarkable induction of apoptosis and senescence was also obtained in TRF2 ΔBΔM -expressing cells, whereas 2′- O -MeRNA treatment did not show these effects. The induction of apoptosis and accelerated senescence has been described as one of the characteristics of G-quadruplex-interacting ligands in cancer cells [30] , [38] , [39] , [45] . To address the molecular mechanism associated with growth arrest and accelerated senescence induced by SWNTs, immunoblots were performed to investigate changes in the expression of p21 and p16 proteins [30] , which have been considered as key regulators of cell cycle and cellular senescence [30] , [35] . As indicated in Fig. 7d , after 3 weeks exposure to SWNTs (50 μg ml −1 ), significant upregulation of p16 and p21 was observed in both K562 and HeLa cells, indicating that p16 and p21 were involved in the growth inhibition. In the same manner, TRF2 ΔBΔM expression also induced obvious upregulation of p16 and p21, whereas 2′- O -MeRNA did not. The involvement of p16 and p21 in telomere-directed senescence has been sufficiently validated [35] . Furthermore, the cell proliferation defects induced by low level of SWNTs over long time incubation have also been demonstrated. As shown in Supplementary Figure S13 and S14 , over long-time treatment (almost 2 months), low level of SWNTs accumulated in cells and growth arrest occurred, which was dependent on the persistence of SWNTs in the medium, and the total telomere erosion induced by the continual telomerase activity inhibition. Compared with G-quadruplex, the biological relevance of i-motif structure has not been fully understood. In this report, we demonstrate that stabilization of i-motif DNA by SWNTs can inhibit telomerase activity both in vitro and in vivo , and induce telomere uncapping, leading to removal of telomere-binding protein from telomere, and production of DNA-damage response and subsequent cell growth cessation. Even if i-motif may not be expected to directly inhibit telomerase, their formation could make the complementary G-rich DNA to form G-quadruplexes in telomeres just as those found in the promoters of certain oncogenes [8] , [46] , [47] . As many G-quadruplex-interactive ligands can stabilize G-quadruplex [39] , [45] , [48] , [49] , the formed G-quadruplex would inhibit telomerase activity and block telomere elongation. It should be pointed out that the precise mechanism for SWNTs-induced intracellular telomerase inhibition and the consequent events remains not completely understood. Continued studies are worthy of detailed investigation, such as the long-term effects on telomerase, telomere and telomeric proteins essential for end-capping [50] , such as TRF2, POT1. As many other G-/C-rich regions in the human genome that can adopt i-motif/G-quadruplex structures, especially in the promoter regions of many genes and at recombination hotspots [8] , [36] , although SWNTs have relatively high specificity for telomeric DNA, they may also affect expressions of other genes, which are related to regulation of telomerase activity [8] , [46] , [51] . Therefore, telomerase inhibition may have involved mutiple cross-talks between them. Telomeric quadruplex formation induced by SWNTs has resulted in the removal of telomere-binding proteins TRF2 and POT1 from telomere, which has been identified to have important roles in telomere maintenance and end-protection [1] , [34] , [35] . The reason for that SWNTs do not affect another telomeric dsDNA-binding protein, TRF1 binding to telomere may be due to its different binding sites from TRF2 on telomere and different roles. TRF1 has a propensity for binding long tracts of dsDNA and has been postulated to modulate the length of telomere via its interaction with other telomere associated proteins [1] , [50] . In contrast, TRF2 can directly bind not only the telomeric dsDNA but also the ds/ssDNA junction near the 3′-overhang, and promote the overhang to invade the upstream duplex region to form the T-loop structure [1] , [3] , [52] . Moreover, TRF1 has been reported to have an approximately four times higher binding affinity to telomeric DNA than TRF2 [53] . Therefore, when the telomeric DNA forms quadruplex structure, TRF2 would be more sensitive and easily to dissociate from telomere than TRF1. PCBP1 protein has been identified as the most specific binding protein for telomeric C-rich DNA and may be presented in the human telomere–telomerase complex [42] , [43] . We also observed removal of PCBP1 protein from telomere after treatment with SWNTs. However, up to now, the real mechanism for PCBP1 protein on telomere regulation has not been fully illustrated [54] , and substantial works are currently needed. Our confocal microscope, ChIP and reciprocal IP results demonstrate that PCBP1 can localize at telomere and interact with TRF1 and TRF2 proteins ( Fig. 6 and Supplementary Figs S15 and S16 ), which may suggest PCBP1 possibly involved in telomere maintenance. Moreover, the removal of PCBP1, a specific telomeric C-rich DNA-binding protein, provides the indirect evidence for the formation of i-motif induced by SWNTs in vivo , just as those observed in the promoters of some oncogenes [46] , [47] , [55] . Previous studies have demonstrated that quadruplex formation at telomere and concomitant telomere uncapping can activate some nucleases/exonucleases to process the ends, which result in rapid reduction of telomeric G-overhang signals [14] , [56] , [57] ; removal of telomere-binding proteins (TRF2 and POT1) from telomere can also cause loss of telomeric G-overhang [1] , [34] , [37] , [38] ; the slight reduction of G-overhang induced by transfection with 2′- O -MeRNA may indicate that the length of telomeric 3′-overhang is proportional to the rate of telomere shortening in human cells [58] , [59] . Therefore, based on these facts and our results, SWNTs can bind at telomere, inhibit telomerase activity and trigger a series of telomere-related cellular events, following the similar way as G-quadruplex-binding ligands [30] , [37] , [38] , [39] ( Fig. 8 ). This is the first example that stabilization of i-motif structure can inhibit telomerase activity and interfere with the telomere functions in cancer cells. Our work provides new insights into understanding the biomedical effects of SWNTs in cancer cells and the biological importance of i-motif structure in vivo . 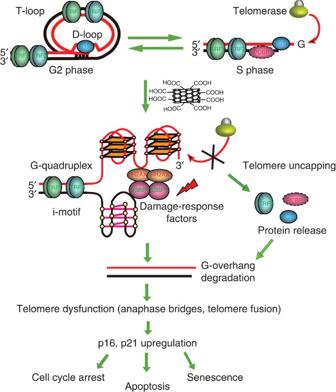Figure 8: Schematic illustration of the telomerase inhibition and telomere uncapping induced by carboxylated SWNTs. The telomere is postulated to form a lariat-like structure, in which the 3′-G-overhang of the telomere invades a duplex telomeric region to form a double-stranded T-loop and a single-stranded D-loop. During DNA replication, the 3′-overhang becomes accessible to telomerase to elongate telomeres. However, in the presence of carboxylated SWNTs, the C-rich telomeric strand self-assemble into an i-Motif structure, whereas the corresponding complementary G-rich strand adopts compact G-quadruplex, resulting in the block of telomere elongation by telomerase. The persistence of i-motif and G-quadruplex would lead to telomere uncapping and disrupt the telomeric loop structure, resulting in formation of anaphase bridges and telomere fusion, characteristics of telomere dysfunction. SWNTs also induce release of telomere-binding protein (TRF2, POT1 and PCBP1) from telomere and cause the degradation of telomeric 3′-overhang. The dysfunctional telomere elicits DNA damage response at telomeres and activates the DNA repair pathways, resulting in p16, p21-mediated cell cycle arrest, apoptosis and senescence to suppress further growth of genomically unstable cells. Figure 8: Schematic illustration of the telomerase inhibition and telomere uncapping induced by carboxylated SWNTs. The telomere is postulated to form a lariat-like structure, in which the 3′-G-overhang of the telomere invades a duplex telomeric region to form a double-stranded T-loop and a single-stranded D-loop. During DNA replication, the 3′-overhang becomes accessible to telomerase to elongate telomeres. However, in the presence of carboxylated SWNTs, the C-rich telomeric strand self-assemble into an i-Motif structure, whereas the corresponding complementary G-rich strand adopts compact G-quadruplex, resulting in the block of telomere elongation by telomerase. The persistence of i-motif and G-quadruplex would lead to telomere uncapping and disrupt the telomeric loop structure, resulting in formation of anaphase bridges and telomere fusion, characteristics of telomere dysfunction. SWNTs also induce release of telomere-binding protein (TRF2, POT1 and PCBP1) from telomere and cause the degradation of telomeric 3′-overhang. The dysfunctional telomere elicits DNA damage response at telomeres and activates the DNA repair pathways, resulting in p16, p21-mediated cell cycle arrest, apoptosis and senescence to suppress further growth of genomically unstable cells. Full size image Chemical modification of CNTs SWNTs ( =1.1nm, purity >90%) were purchased from Aldrich (St Louis, MO, USA) and MWNTs ( =10–20 nm) were purchased from Nanotech Port Co. Ltd. (Shenzhen, China). The preparation and characterization (size and surface charges) of chemically modified CNTs have been described in detail in previous reports [11] , [12] , [13] , [14] , [15] , [16] , [17] , [18] , [32] . In brief, the carboxyl-modified CNTs (SWNT-COOH, MWNT-COOH) were prepared by sonicating the primitive CNTs in a 3:1 v/v solution of concentrated sulfuric acid (98%) and concentrated nitric acid (70%) for 24 h at 35–40 °C and washed with water, leaving an open hole in the tube side and functionalized the open end of CNTs with carboxyl groups to increase their solubility in aqueous solution. The hydroxyl-modified SWNTs (SWNT-CH 2 OH) were obtained by reducing carboxyl-modified SWNTs, using lithium aluminum hydride (LiAlH 4 ) in anhydrous tetrahydrofuran. After reduction, samples were successively washed with methanol, diluted HCl and water. The ethylenediamine-modified SWNTs (SWNT-CONHCH 2 CH 2 NH 2 ) were synthesized by a routine method [11] , [12] , [16] , suspending the carboxyl-modified SWNTs in thionyl chloride (SOCl 2 ) solution containing 5% dimethylformamide, and circle heating for 24 h at 70 °C, then washing with tetrahydrofuran. Acyl chloride-modified SWNTs (SWNT-COCl) were obtained. These CNTs were then mixed with ethylenediamine, stirred for 96 h, followed by washing with ethanol and dichloromethane; ethylenediamine-modified SWNTs were obtained by amide bond formation. The characterizations of different functionalized CNTs were summarized in Supplementary Methods . Carboxyl-modified SWNTs were further used to attach aminopolymers polyethylene glycol (PEG 1500N ) to the nanotubes via amide linkages [27] . The PEG-SWNTs were then labelled with fluorescent dye FITC to facilitate biological imaging. Detailed information on the preparation and characterization of SWNT samples was described in Supplementary Methods . Cell culture and agents Human chronic myelogenous leukemia K562 cells and human cervical carcinoma HeLa cells were grown in Iscove's modified Dulbecco's medium (Gibco BRL) supplemented with 10% FCS in a humidified 37 °C incubator with 5% CO 2 . Exponentially growing cells were used for the experiments. 2′-O-methyl-RNA with a phosphorothioate (ps) backbone (5′-2′-O-methyl [C(ps)A(ps)GUUAGGGUU(ps)A(ps)G]-3′), obtained from TaKaRa, were dissolved in sterile water, aliquoted and stored at −20 °C until further processing. Cell-free telomerase assay (TRAP-G4) The ability of agents to inhibit telomerase in a cell-free assay was assessed with a TRAP assay [28] . A modified TRAP-G4 was also used for G-quadruplex-induced telomerase activity assay [20] , [21] , [22] , [23] . A mimic of telomeric duplex DNA (5′-AG 3 (T 2 AG 3 ) 3 GTTAGT-3′ (G-DNA):5′-(C 3 TA 2 ) 3 C 3 T-3′(C-DNA)) with a 6-nt of 3′-tail (underlined) was first created by mixing equimolar amounts of each strand (0.4 μM per strand) in 1×TKG buffer (50 mM Tris-HCl (pH 8), 60 mM potassium glutamate), heating to 90 °C for 5 min, and slow-cooling to room temperature. Then it was extended by telomerase in a volume of 44 μl containing 20 mM Tris–HCl (pH 8.3), 100 μM dNTP, 1.5 mM MgCl 2 , 63 mM KCl, 1 mM EGTA, 0.005% Tween 20, 100 μg ml −1 BSA, 5 μl telomerase crude extract prepared from K562 cells, and various concentrations of CNTs. After 30-min incubation at 30 °C, the reaction was terminated by heating at 94 °C for 5 min, followed by addition of 6 μl PCR mixture containing 8.3 pmol of primers TS (5′-AATCCGTCGAGCAGAGTT-3′) and NT (5′-ATCGCTTCTCGGCCTTTT-3′), 1 amol of TSNT (5′-AATCCGTC GAGCAGAGTTAAAAGGCCGAGAAGCGAT-3′) template for internal standard and 1 U of Taq DNA polymerase (Ex Taq Hot Start, TaKaRa). The samples were subjected to 30 PCR cycles of 94 °C for 30 s, 55 °C for 30 s and 72 °C for 90 s. Ten microlitre PCR products were resolved on 12% polyacrylamide gel, stained with 0.2% AgNO 3 and recorded on a UVP gel documentation system (Ultraviolet Products, Upland, CA, USA). Telomerase activity was assessed by determining the ratio of the entire telomerase ladder to that of the internal control, using Lab works 4.5 image analysis software. Cell-based telomerase assay Cells were seeded on six-well plates (1.0×10 5 per well) and pre-incubated for 24 h at 37 °C in a humidified atmosphere of 5% CO 2 before exposure to various dilutions of CNTs. After washing with PBS, crude cell extracts were prepared and total protein concentrations were determined with Bradford assay. Using equivalent total protein amounts (500 ng), telomerase activity in each extract was determined by conventional TRAP assay [28] ; the telomerase products quantified and normalized to the internal standard. Construction and transfection of expression plasmids pLPC-NMYC-TRF2ΔBΔM were taken as the template plasmids, which was obtained from Addgene (plasmid 16069, de Lange Titia, Rockfeller University). The TRF2 ΔBΔM gene was amplified by PCR with primers containing Eco RI and Bam HI sites and cloned into the corresponding cloning sites in the pcDNA3.1/myc mammalian expression vector. The plasmids were transfected with Lipofectamine 2000 (Invitrogen) following the manufacturer's instruction. Forty-eight hours after transfection, positive transfected cells were selected with 600 μg ml −1 G418. The Myc tag was detected by western blotting. Cell proliferation assay Cells were seeded in growth medium into T80 tissue culture flasks at 1.25×10 5 cells per flask and exposed to 25 and 50 μg ml −1 carboxylated SWNTs, respectively, or transfected with 2′- O -methyl-RNA using Lipofectamine 2000, as described above, every 3 days. The cells in control and CNTs-treated flasks were trypsinized and counted using a hematocytometer, and the flasks were reseeded with 1.25×10 5 cells per flask. For cells stably expressing TRF2 ΔBΔM , same concentrations of cells were seeded, and every 3 days, the cells were trypsinized and counted, and flasks were reseeded with the same number of cells. Results were expressed as the cumulated population doubling as a function of the time of culture as described previously [18] , [30] . ChIP assays ChIP assays were performed according to manufacture's instructions (Millipore). Briefly, cells were fixed in 0.8% paraformaldehyde in 1×PBS, washed extensively in 1×PBS, lysed in ice-cold Lysis buffer (1% SDS, 10 mM EDTA, 50 mM Tris–HCl at pH 8.0 and protease inhibitors; sonicated chromatin products of ~100–300 bp) and diluted 10× in dilution buffer (20 mM Tris–HCl at pH 8.0, 150 mM NaCl, 2 mM EDTA, protease inhibitors and 1 mg ml −1 BSA). ChIP was performed with the relevant antibody and captured with Protein A/G-Sepharose. DNA–protein complex was washed with 1× wash buffer I (20 mM Tris-HCl at pH 8.0, 150 mM NaCl, 0.1% SDS, 1% Triton X-100 and 2 mM EDTA), 2× wash buffer II (20 mM Tris–HCl at pH 8.0, 250 mM NaCl, 0.1% SDS, 1% Triton X-100 and 2 mM EDTA) and eluted in 1% SDS and 100 mM NaHCO 3 . Eluate fraction was de-cross-linked by high-salt treatment (200 mM NaCl) at 60 °C followed by proteinase K treatment at 50 °C. DNA extracted was subjected to PCR (see below). Standard and telomere PCR analysis Telomeric sequences in immunoprecipitates were evidenced by PCR amplification according to a method described previously [37] . The final telomere primer concentrations were 270 nM (tel1) and 900 nM (tel2), and PCR amplification was subjected to 35 cycles of 95 °C for 15 s, 54 °C for 2 min. The primer sequences were as following: tel1 5′-GGTTTTTGAGGGTGAGGGTGAGGGTGAGGGTGAGGGT-3′ and tel2 5′-TCCCGACTATCCCTATCCCTATCCCTATCCCTATCCCTA-3′. Quantitative PCR was done using the SYBR green Jumpstart Taq ReadyMix (TaKaRa) on a Roche LightCycler 480. G-tail telomere HPA For HPA [38] , [44] , 1 μg non-denatured genomic DNA and 0.5 μg heat-denatured genomic DNA was used per assay for the detection of telomere 3′ overhangs and total telomere DNA, respectively. Briefly, 100 μl of 3×10 6 rlu (relative light units) of acridiniumester (AE)-labelled telomere HPA probe (5′-CCCTAACCCTAAC C CTAACCCTAACCCTA-3′; AE position is underlined) in hybridization buffer was added to the DNA solution, mixed well by vortex and incubated at 60 °C for 20 min. Specific activity of AE-labelled probe was 8×10 7 rlu pmol −1 probe DNA. Hydrolysis of the AE of unhybridized probes was carried out by adding 300 ml of the hydrolysis buffer to each reaction tube, mixing well by vortex and incubating at 60 °C for 10 min. The AE of hybridized probe was not hydrolysed under these conditions. The tubes were cooled on ice for over 1 min, and chemiluminescence was measured for 2 s per tube with a luminometer (BPCL-2-TGC, Ultra Weak Luminescence Analyzer). For normalization of genomic DNA amount in each assay, we used Alu repetitive HPA probe (5′-TGTAATCCC A GCACTTTGGGAGGC-3′; AE position is underlined). To check specificity of G-tail detection, non-denatured genomic DNA was treated with Exonuclease I (30 U μg −1 DNA) at 37 °C for overnight and heat inactivated at 80 °C for 20 min before G-tails were assayed. Probes for AE-labelling of telomeres and detection of Alu sequences were supplied by Bioneer Inc (Korea). Telomere TdT assay Labelling unprotected telomeres with cy3-conjugated deoxy-Uridine (Amersham) was performed essentially as described [41] , except that the TdT incubation time was 20 min at 37 °C to minimize background. Co-localization of the TdT signal with telomeres was performed by fixing TdT-labelled cells with 2% paraformaldehyde, washing three times in PBS, followed by incubation with anti-TRF1 antibody, and visualized with fluorescein-conjugated secondary antibody. Images were taken using an Olympus Fluoview FV1000 confocal microscope. Statistical analysis The data were expressed as means±s.d. Statistical analysis was performed by Student's t- test (one- or two-tailed). The criterion for statistical significance was taken as P <0.05 or P <0.01. Other related experimental methods, such as semi-quantitative RT–PCR, immunofluorescence, immunoblotting, cytogenetic analysis, cell cycle, apoptosis, senescence, immunuprecipitation and telo-FISH and so on are available in Supplementary Methods . How to cite this article: Chen, Y. et al . Insights into the biomedical effects of carboxylated single-wall carbon nanotubes on telomerase and telomeres. Nat. Commun. 3:1074 doi: 10.1038/ncomms2091 (2012).